Mitotic catenation is monitored and resolved by a PKCε-regulated pathway Exit from mitosis is controlled by silencing of the spindle assembly checkpoint (SAC). It is important that preceding exit, all sister chromatid pairs are correctly bioriented, and that residual catenation is resolved, permitting complete sister chromatid separation in the ensuing anaphase. Here we determine that the metaphase response to catenation in mammalian cells operates through PKCε. The PKCε-controlled pathway regulates exit from the SAC only when mitotic cells are challenged by retained catenation and this delayed exit is characterized by BubR1-high and Mad2-low kinetochores. In addition, we show that this pathway is necessary to facilitate resolution of retained catenanes in mitosis. When delayed by catenation in mitosis, inhibition of PKCε results in premature entry into anaphase with PICH-positive strands and chromosome bridging. These findings demonstrate the importance of PKCε-mediated regulation in protection from loss of chromosome integrity in cells failing to resolve catenation in G2. The metaphase-to-anaphase transition is the critical point in the cell cycle where the cell commits to separation of sister chromatids. Mistakes at this stage can lead to aneuploidy and chromosome breakages, which are features common in cancer [1] . Before anaphase, spindle assembly checkpoint (SAC) monitors correct spindle attachment and biorientation of sister chromatids [2] . Once spindle attachment is complete, cohesion must be eliminated to enable the physical separation of sister chromatids. This requires cleavage of the protein complex cohesin by separase and, in some instances, completion of chromosome decatenation [3] , [4] , [5] , [6] , [7] . Loss of topoisomerase activity in metaphase leads to delayed exit and extensive anaphase chromosome bridging, often resulting in cytokinesis failure, although maintenance of limited catenation until anaphase may be important for sister chromatid structural organization [8] , [9] , [10] . Anaphase is initiated by activation of an E3 ubiquitin ligase complex, the anaphase promoting complex (APC), which directs protease-mediated degradation of anaphase inhibitors cyclinB1 and securin [11] . Various mitotic signalling components are transiently localized to the kinetochore during mitosis and control of their dynamic association with the kinetochore generates a diffusible inhibitor of the APC [11] , [12] . This inhibitory complex is maintained until bioriented microtubule engagement is established for all sister chromatid kinetochores. Kinetochore signalling components include the checkpoint proteins Bub1, BubR1 and Mad2 (ref. 13 ). Other regulatory components present at the kinetochore include the RZZ complex (Rod, ZW10, Zwilch) [14] and various motor proteins including dynein and CENP-E [15] , [16] . Once all sister chromatids are bioriented, the APC is activated and anaphase is initiated. SAC silencing is a complex process and various mechanisms are involved in regulating anaphase onset. These include the activation of PP1 phosphatase activity [17] , [18] , [19] , ubiquitination of cdc20 by the APC [20] and dynein-mediated streaming of checkpoint components from the kinetochore, a process which is regulated by the RZZ complex [21] , [22] . Regulation of mitotic exit when biorientation is incomplete is well studied [23] , but how anaphase is delayed when sister chromatids retain catenation is unclear. DNA catenanes formed during replication are corrected by topoisomerase II (topoII), which is essential for complete decatenation of sister chromatids and subsequent segregation in mitosis [24] . Topoisomerase IIa (topoIIa) is associated with mitotic chromosome arms throughout mitosis [25] and plays an essential role in mouse embryonic development as disruption of the topoIIa gene is lethal at the four- to eight-cell stage where cells show evidence of mitotic segregation failures [26] . Consistently, either inhibition of topoIIa using bis(2,6-dioxopiperazine) derivatives such as ICRF193 or depletion of topoIIa in human cells results in anaphase chromosome bridging, leading to polyploidy and cell death [8] , [27] . Persistence of DNA sister chromatid catenation during anaphase is likely to promote DNA damage and genomic instability through chromosome non-disjunction and breakage [28] . Thus, topoIIa-mediated decatenation of sister chromatids is required for proper cell division. A catenation-sensitive delay at the metaphase-to-anaphase transition has been identified in both vertebrates [4] , [29] , [30] , [31] and budding yeast [32] . However, there are few insights into what signalling molecules are involved in this process and what relationship this has with the SAC. Here we demonstrate that protein kinase Cε (PKCε) controls a pathway required to trigger and maintain the catenation-dependent metaphase delay characterized by retention of a subset of SAC regulators. This delay can be overridden without catenation resolution by PKCε ablation or inhibition, thus representing a metaphase control point rather than a physical block to anaphase onset. Using a direct measure of metaphase catenation, we demonstrate that this PKCε pathway controls catenation resolution in mitosis. We thereby show that PKCε becomes engaged when there is excess metaphase catenation, and that it controls a pathway that delays anaphase entry and promotes decatenation. We and others have identified transformed cell lines that have a leaky G2 catenation checkpoint [33] . We hypothesize that this process acts as a failsafe mechanism to protect cells that aberrantly enter mitosis with excess catenation. Importantly, we find that non-transformed cells with a robust G2 catenation arrest do not enter mitosis with catenated sister chromatids and display no dependence on the PKCε-regulated pathway, suggesting a potentially excellent therapeutic index for PKCε intervention in cancer. PKCε regulates mitotic catenation resolution We have reported previously that PKCε is important in completion of cytokinesis [34] , [35] . Here we imaged HeLa cells by time-lapse microscopy and found evidence of an earlier mitotic defect as a result of PKCε loss, which manifests as an increase in anaphase chromosome bridging, demonstrated by an increase in the mean number of anaphase chromosome bridges by 55.7% (siControl versus PKCε si1, P =0.0008; Fig. 1a,b ). We observe heterogeneity between the three different small interfering RNAs (siRNAs) used and attribute this to efficiency of knockdown ( Fig. 1a ). The chromatin bridging typically consists of large sections of chromatin emanating from both sides of the furrow, often with a central section that is not marked by mCherry-H2B or 4',6-diamidino-2-phenylindole (DAPI; Fig. 1b,c ). We inspected these structures by correlative light and electron microscopy (CLEM) and found that the large chromatin sections were linked together by thin stretches of DNA, which are continuous through the furrow ( Fig. 1c ). The mitotic spindle appears to be correctly attached at the kinetochore as the centromeres segregate normally, indicating that the bridging portions do not represent incorrect kinetochore attachments ( Fig. 1d ). Anaphase chromatin bridging persisted into telophase in 61.5% of telophase cells scored and the centromere section of the chromosome was not seen in the furrow ( Supplementary Fig. 1a ). Intriguingly, we did not see any such chromatin bridging in normal diploid RPE-1 cells after knockdown of PKCε ( Supplementary Fig. 1b ). 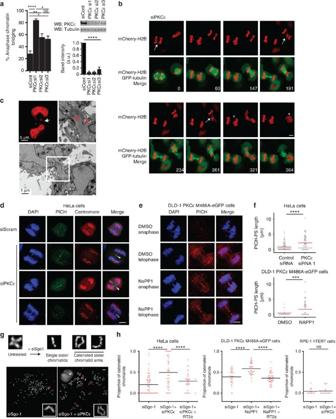Figure 1: Knockdown of PKCε causes chromatin bridging that is associated with an increase in both metaphase and anaphase catenation. (a–c) HeLa cells that stably express mCherry-H2B and GFP-Tubulin (HeLa H2B) were imaged by time-lapse microscopy. (a) Graph showing the number of HeLa-H2B cells that enter anaphase with chromatin bridging. Cells were treated with either control siRNA or one of three different siRNAs that target PKCε (si1, si2 and si3) and imaged by time-lapse microscopy. Graph shows average of three experiments±s.e.m.,n>30 per experiment, per condition. Right panel shows quantification of knockdown to show correlation between knockdown and the frequency of chromatin bridges observed, chart shows mean ±s.d. (n=3) (b) Stills taken from time-lapse imaging of HeLa-H2B cells after treatment with PKCε si1; time in minutes marked in white. (c) CLEM image of a Hela H2B cell in cytokinesis showing chromatin in red (arrowed) and juxtaposed electron micrograph sections showing details of this chromatin bridge. Top right panel shows a higher magnification of the area denoted by the white box in the far right panel, the red arrow shows electron dense chromatin bridges. (d) Immunoflourescence images of HeLa cells after treatment±PKCε siRNA showing PICH-PS (green), centromeres by ACA staining (red) and DAPI (blue). Open arrows indicate PICH-positive strands that do not colocalize with DAPI, and closed arrows indicate PICH and DAPI colocalization, stared open arrow indicates DAPI-positive bridges with no PICH staining. (e,f) PICH-PS are more persistent after PKCε knockdown or inhibition evidenced by long PICH-PS. Immunoflourescence images of DLD-1 PKCε M486A cells after treatment with NaPP1showing examples of PICH-PS that are persistent into telophase PICH-PS (red) and DAPI (blue). (f) Chart shows length of PICH-PS measured using Zen software (Zeiss), red line indicates mean length, each spot represents a single strand (n>70). (g, upper panel) Scheme to describe the basis of the catenation spread assay. (g, lower panel) Representative example images of catenation spread assay with catenated sister chromosomes starred and an example chromosome enlarged for clarity. (h) Chart shows the percentage of sister chromatids per cell with catenated chromosomes; mean shown by black line (n>30 cells, repeated three times). Scale bars, 5 μm (unless otherwise stated). Figure 1: Knockdown of PKCε causes chromatin bridging that is associated with an increase in both metaphase and anaphase catenation. ( a – c ) HeLa cells that stably express mCherry-H2B and GFP-Tubulin (HeLa H2B) were imaged by time-lapse microscopy. ( a ) Graph showing the number of HeLa-H2B cells that enter anaphase with chromatin bridging. Cells were treated with either control siRNA or one of three different siRNAs that target PKCε (si1, si2 and si3) and imaged by time-lapse microscopy. Graph shows average of three experiments±s.e.m., n >30 per experiment, per condition. Right panel shows quantification of knockdown to show correlation between knockdown and the frequency of chromatin bridges observed, chart shows mean ±s.d. ( n =3) ( b ) Stills taken from time-lapse imaging of HeLa-H2B cells after treatment with PKCε si1; time in minutes marked in white. ( c ) CLEM image of a Hela H2B cell in cytokinesis showing chromatin in red (arrowed) and juxtaposed electron micrograph sections showing details of this chromatin bridge. Top right panel shows a higher magnification of the area denoted by the white box in the far right panel, the red arrow shows electron dense chromatin bridges. ( d ) Immunoflourescence images of HeLa cells after treatment±PKCε siRNA showing PICH-PS (green), centromeres by ACA staining (red) and DAPI (blue). Open arrows indicate PICH-positive strands that do not colocalize with DAPI, and closed arrows indicate PICH and DAPI colocalization, stared open arrow indicates DAPI-positive bridges with no PICH staining. ( e , f ) PICH-PS are more persistent after PKCε knockdown or inhibition evidenced by long PICH-PS. Immunoflourescence images of DLD-1 PKCε M486A cells after treatment with NaPP1showing examples of PICH-PS that are persistent into telophase PICH-PS (red) and DAPI (blue). ( f ) Chart shows length of PICH-PS measured using Zen software (Zeiss), red line indicates mean length, each spot represents a single strand ( n >70). ( g , upper panel) Scheme to describe the basis of the catenation spread assay. ( g , lower panel) Representative example images of catenation spread assay with catenated sister chromosomes starred and an example chromosome enlarged for clarity. ( h ) Chart shows the percentage of sister chromatids per cell with catenated chromosomes; mean shown by black line ( n >30 cells, repeated three times). Scale bars, 5 μm (unless otherwise stated). Full size image PICH (Plk-1 checkpoint helicase) binds to fine strands of DNA that span the anaphase plate and are postulated to be associated with centromeric catenated DNA [36] . As we observed fine strands of DNA in the furrow by CLEM ( Fig. 1c ), we employed PICH as a marker of ultra-fine strands, to quantify the association between loss of PKCε and the appearance of these strands. We indeed saw a change in PICH-positive strands (PICH-PS) after PKCε knockdown, which increased from 25% of cells in the control to 64% in cells treated with PKCε si1 ( Fig. 1d ). This high basal level of PICH-PS in control cells is corroborated by others [37] . We confirmed this finding in a second cell line and exploited the PKCε M486A gatekeeper mutant. The small molecule NaPP1 binds to very few wild-type kinases due to a steric clash with the gatekeeper residue in the ATP-binding pocket; PKCεM486A is inhibited, as the gatekeeper residue has been substituted with a less bulky alanine [35] , [38] . In the DLD-1 PKCεM486A cell line, we observe an increase in PICH-PS from 16% under basal conditions to 58% in cells after treatment with NaPP1. These PICH-PS generally did not co-localize with the DAPI-stained chromatin bridges (23% colocalization in HeLa and 25% colocalization in DLD-1 PKCεM486A cells; see Fig. 1d,e ), indicating that most of the PICH-PS can be attributed to ultra-fine stretches of DNA as seen by others [7] , [36] , [37] , [39] . In addition to an increase in the number of PICH-PS, we also observe an increased persistence of these strands into late anaphase and telophase, and this manifests as very long PICH-PS after PKCε inhibition or knockdown ( Fig. 1e,f ). Chromosome bridging and PICH-PS have been associated with an increase in anaphase catenation [7] , [36] , [37] , [39] , [40] , we therefore investigated whether the increase in chromosome bridging seen after PKCε knockdown correlates with an increase in metaphase catenation. DNA catenation in mitosis can trigger a delayed exit from mitosis [29] , [30] , [31] and there may be a varying requirement in different cell lines for decatenation in metaphase, dependent on the fidelity of the G2 catenation checkpoint [41] , [42] . We therefore sought to establish the cause of the anaphase bridging that we observed on PKCε knockdown. We hypothesized two non-exclusive scenarios: (i) that there may be a high basal level of metaphase catenation in these cell lines, which is inefficiently resolved due to the loss of a PKCε-promoted decatenation pathway or (ii) that PKCε may operate a checkpoint-associated response to metaphase catenation, which would normally implement a metaphase delay, providing time for decatenation and preventing bridging in anaphase. To address whether there is an increase in mitotic catenation, we directly measured the degree to which sister chromatids were catenated in prometaphase. In this assay, we monitor sister chromatid catenation by enabling the removal of centromeric cohesin and then viewing the chromosome formations. Centromeric cohesion is protected from removal during prophase by Sgo-1 (ref. 43 ). When Sgo-1 is targeted, sister chromosome cohesion is lost resulting in mitotic cells with single sister chromatids. The extent to which sister chromatids are catenated is revealed as a tethering of sister chromatid arms ( Fig. 1g and Supplementary Fig. 2 ). The frequency of this tethering increases with knockdown of topoIIa by siRNA as expected ( Supplementary Fig. 2 ), and in confirmation that the structures seen here reflect catenation, we found that addition of recombinant topoIIa ex vivo reversed the tethering phenotype observed ( Fig. 1h ). We applied this assay to determine whether PKCε plays a role in metaphase decatenation. Interestingly, we saw an increase in metaphase catenation after PKCε knockdown using siRNA ( Fig. 1g,h ) and this could be recovered using recombinant topoIIa, suggesting that the tethering seen in this assay represents catenation. We confirmed this using the DLD-1 PKCεM486A cell line and find that specific inhibition using NaPP1 also caused an increase in sister chromatid catenation in metaphase ( Fig. 1h ) In contrast to our findings above in the HeLa and DLD-1 cells, PKCε knockdown in the non-transformed RPE-hTERT cells did not increase either metaphase catenation or PICH-PS ( Fig. 1h ) and, in fact, out of over 100 fields of view revealing at least 30 early anaphase cells, we did not see any PICH-PS. This is in line with our observation that we also do not see an influence of PKCε on chromatin bridging in RPE-1 cells ( Supplementary Fig. 1b ). We did observe an increase in metaphase catenation after TopoIIa knockdown in this cell line, which is expected, as TopoIIa is essential for both decatenation and arrest at the G2 catenation checkpoint [44] , [45] . We could not rescue this increase in catenation, as it was much more pronounced than the other two cell lines. Given this evidence, we hypothesized that the PKCε-dependent phenotype seen in HeLa and DLD-1 cells may be due to a requirement for a metaphase decatenation pathway in response to excess catenation persisting from G2. To investigate the possible G2 origin of the metaphase catenation, we carried out a fluorescence-activated cell sorting (FACS) analysis to compare the robustness of the G2 checkpoint in the three cell lines discussed above. We used ICRF193 to assay the G2 checkpoint response to catenation and bleomycin to measure the checkpoint response to DNA damage [41] , [46] . In line with our previous observations, RPE1-hTERT arrest robustly in G2 when treated with either ICRF193 or bleomycin ( Fig. 2a,b ). This could be weakened using an Ataxia telangiectasia mutated/ATM-RAD3-related inhibitor as expected. Both HeLa and DLD-1 cells had a more leaky response to either ICRF193 or bleomycin, indicating that they both have a weakened G2 catenation checkpoint as predicted. 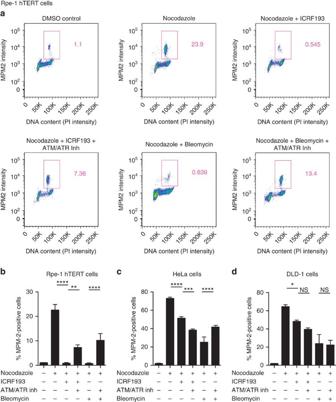Figure 2: RPE-1 hTERT cells have an intact G2 checkpoint but this response is weak in HeLa and DLD-1 cells. (a) RPE-1 hTERT cells have a robust G2 checkpoint shown by FACS analysis. Cells were treated for 24 h with the indicated inhibitors and analysed by FACS. Scatter charts show DNA content plotted against MPM-2 intensity to measure the number of cells that escape the G2 checkpoint into a nocodazole arrest in mitosis. The percentage of MPM-2-positive cells was analysed and plotted inb–dfor the three different cell lines as indicated (chart shows average of three experiments ±s.e.m.,n>10,000 cells counted per condition). Figure 2: RPE-1 hTERT cells have an intact G2 checkpoint but this response is weak in HeLa and DLD-1 cells. ( a ) RPE-1 hTERT cells have a robust G2 checkpoint shown by FACS analysis. Cells were treated for 24 h with the indicated inhibitors and analysed by FACS. Scatter charts show DNA content plotted against MPM-2 intensity to measure the number of cells that escape the G2 checkpoint into a nocodazole arrest in mitosis. The percentage of MPM-2-positive cells was analysed and plotted in b – d for the three different cell lines as indicated (chart shows average of three experiments ±s.e.m., n >10,000 cells counted per condition). Full size image PKCε is required to trigger the metaphase catenation delay Excessive catenation in mitosis causes a delay to anaphase entry [29] , [30] , [31] , and as we see evidence of catenation entering anaphase in our transformed cell lines when PKCε is compromised, we postulated that the metaphase catenation delay may also be abrogated after loss of PKCε. In agreement with Huang et al. [47] , we find that the topoIIa inhibitor ICRF193 triggers a transient metaphase delay of 94±6.6 min ( P <0.0001) in HeLa cells and 119±7.1 min, ( P <0.0001) in DLD-1 cells ( Fig. 3a–d ). In these assays, we use time-lapse microscopy to record images of either DLD-1 or HeLa cells expressing mCherry-Histone2B and record the time taken from metaphase alignment to sister chromatid separation in anaphase. In the presence of ICRF193, the anaphase achieved is very unequal and more difficult to detect as shown in Fig. 3d . This is likely to be due to an excess of catenation preventing sister chromatid separation. Interestingly, we find that this metaphase delay is very dependent on PKCε and using siRNA we see a reduced metaphase delay by 54±7 min ( P <0.0001) in HeLa cells ( Fig. 3a,b ). Consistently, knockdown or inhibition of PKCε in DLD-1 cells also bypasses this metaphase delay and decreases the time spent in mitosis by 58±8 min ( P <0.0001; Fig. 3c,d and Supplementary Fig. 1d ). In addition to using NaPP1 to inhibit PKCε in these assays, we also confirmed the specificity of the PKCε siRNA by recovering the phenotype with an siRNA-resistant PKCε construct. In this system, the metaphase delay is recovered as shown by a decrease in the metaphase transition speed of 56±11 min ( P <0.0001) following tetracycline induction of the siRNA-resistant construct, confirming the specificity of the siRNA phenotype ( Supplementary Fig. 1c ). We also investigated whether both the decatenation pathway and the requirement for PKCε could be triggered after the cells had entered mitosis by inhibiting topoIIa and PKCε once cells enter mitosis. As with the data above, we induce a delay to metaphase exit by adding ICRF193 once cells have entered prophase and this is again lost when PKCε is inhibited. This confirms that these cells require PKCε activity to trigger/maintain a metaphase delay in mitosis ( Supplementary Fig. 1d ). 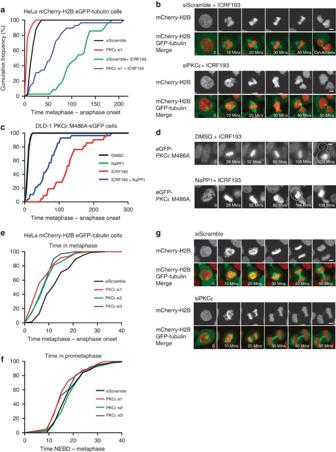Figure 3: Knockdown of PKCε causes cells to enter anaphase prematurely when challenged by catenation. The fidelity of the metaphase catenation arrest was assessed by time-lapse microscopy. (a,b) HeLa-H2B cells were treated for 48 h±siRNA targeting PKCε. Cumulative frequency chart (a) and representative stills, time in minutes marked in white (b) showing time taken in minutes from metaphase-to-anaphase±5 μM ICRF193. (c,d) Inhibition of PKCε M486A in DLD-1 cells abrogates the metaphase catenation delay as illustrated by cumulative frequency chart (c) and representative stills (d), showing time taken in minutes from metaphase to anaphase after treatment with NaPP1±5 μM ICRF193. (e–g) HeLa-H2B cells were treated with either control siRNA or one of three different siRNAs that target PKCε (si1, si2 and si3). (e,f) Cumulative frequency charts showing the time spent in either metaphase (e) or prometaphase (f), and representative stills from the time-lapse videos, time in minutes marked in white (g). For all live-cell experiments,n>30, all experiments repeated three times. Scale bars, 5 μm. Figure 3: Knockdown of PKCε causes cells to enter anaphase prematurely when challenged by catenation. The fidelity of the metaphase catenation arrest was assessed by time-lapse microscopy. ( a , b ) HeLa-H2B cells were treated for 48 h±siRNA targeting PKCε. Cumulative frequency chart ( a ) and representative stills, time in minutes marked in white ( b ) showing time taken in minutes from metaphase-to-anaphase±5 μM ICRF193. ( c , d ) Inhibition of PKCε M486A in DLD-1 cells abrogates the metaphase catenation delay as illustrated by cumulative frequency chart ( c ) and representative stills ( d ), showing time taken in minutes from metaphase to anaphase after treatment with NaPP1±5 μM ICRF193. ( e – g ) HeLa-H2B cells were treated with either control siRNA or one of three different siRNAs that target PKCε (si1, si2 and si3). ( e , f ) Cumulative frequency charts showing the time spent in either metaphase ( e ) or prometaphase ( f ), and representative stills from the time-lapse videos, time in minutes marked in white ( g ). For all live-cell experiments, n >30, all experiments repeated three times. Scale bars, 5 μm. Full size image In addition to a dependence on PKCε to trigger a metaphase delay in response to a topoIIa inhibitor, we also see an increase in the basal metaphase transition speed in HeLa cells after knockdown of PKCε using the most efficient siRNA (PKCεsi1) of 5 ±1.1 min ( P <0.0001) compared with the control ( Fig. 3e,f ). We do not observe any difference in the time taken from prometaphase to metaphase, indicating that chromosome congression to the metaphase plate is not affected by PKCε knockdown. We can again recover this phenotype using the siRNA-resistant PKCε construct, indicating that the effect is specific to PKCε ( P <0.005; Supplementary Fig. 1c ). As with decatenation, we do not see PKCε dependence in RPE-1 cells under basal conditions ( Supplementary Fig. 1e ) and as HeLa cells have high levels of metaphase catenation and PICH-PS in anaphase ( Fig. 1h and Supplementary Fig. 2 ), we propose that the increase in basal transition speed is the result of abrogation of a catenation delay that is routinely engaged by HeLa cells having a ‘leaky’ G2 catenation checkpoint. These results together suggest that the catenation resolution pathway and the arrest triggered by detection of metaphase catenation may be intrinsically linked, as both are highly dependent on PKCε. We tested whether we could induce a dependence on PKCε in RPE-hTERT cells by weakening the G2 catenation checkpoint, to allow entry of catenated DNA into mitosis. We used an Ataxia telangiectasia mutated/ATM RAD3-related inhibitor [48] and, in line with our findings, this causes cells to enter mitosis even when ICRF193 is present and these cells then arrest in metaphase for an extra 65.5±3.7 min ( P <0.0001) compared with the control ( Supplementary Fig. 1f,g ). In line with our observations in HeLa and DLD-1 cells, this delay is abrogated by PKCε knockdown using siRNA by 19±6.4 min ( P =0.0055), suggesting that RPE cells are also dependent on PKCε if they encounter catenation in mitosis. Involvement of PKCε in other perturbations of the SAC The evidence above suggests that PKCε is involved in modulating exit from metaphase under conditions of catenation stress. To address whether this PKCε control is triggered by other known perturbations of anaphase entry, we assayed mitotic transition times in HeLa cells, DLD1 and RPE-hTERT cells under various conditions that perturb the mitotic spindle. Nocodazole treatment was used to assess the fidelity of the SAC response to unattached kinetochores, the Eg5 inhibitor monastrol was used to assess the SAC response to non-bioriented, monopole spindles [49] . All three cell lines tested maintained a robust SAC arrest after loss of PKCε in response to nocodazole ( Fig. 4a,b and Supplementary Fig. 3a,e ) or monastrol ( Fig. 4a,b and Supplementary Fig. 3a,e ), indicating that PKCε is not required for this aspect of the SAC arrest. Taxol was also used at various concentrations to assess the effect of stabilization of the spindle to different degrees. The SAC arrest was entirely insensitive to PKCε modulation in DLD-1 and RPE-1-hTERT cells, indicating that this SAC trigger is not dependent on PKCε. However, in HeLa cells the arrest was weakened on treatment with PKCε siRNA ( Supplementary Fig. 3c,d ). This one contradictory result indicates that PKCε is not an absolute requirement for taxol-mediated mitotic arrest, but can become engaged in some circumstances. Importantly, PKCε dependence on ICRF193-induced metaphase delay was uniformly robust in the transformed cell lines after treatment with either PKCε siRNA or a PKCε inhibitor, Blu557 (Compound 18 (ref. 50 ), Fig. 3 and Supplementary Fig. 1f,g ). Catenation is therefore the only penetrant trigger for the PKCε-dependent mitotic exit that we have tested. 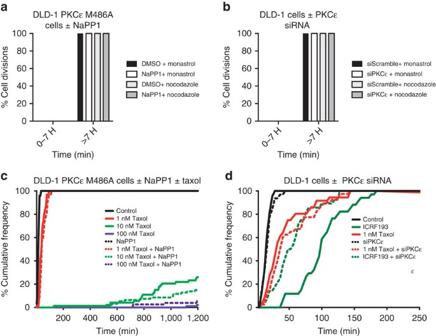Figure 4: Knockdown of PKCε using siRNA does not affect the SAC arrest in DLD-1 cells. (a–d) DLD-1 cells were treated with various SAC triggers and the fidelity of the SAC arrest was measured after loss of PKCε. (a,b) DLD-1 parental cells or DLD-1 PKCε M486A cells were treated with 100 μM Monastrol±20 nM NaPP1 (a) or with PKCε si1 (b) and time taken to transit through mitosis was assayed by time-lapse microscopy by monitoring cell rounding. Charts show the number of cells that maintain a mitotic arrest for more than 7 h. (c,d) DLD-1 parental cells or DLD-1 PKCε M486A cells were treated with taxol or ICRF193 as indicated±20 nM NaPP1 or with PKCε si1 and the time taken to transit through mitosis was assayed by time-lapse video microscopy by monitoring cell rounding. The graph shows the time taken to transit through mitosis as a cumulative frequency chart. For all live-cell experiments,n>30, all experiments repeated three times. Figure 4: Knockdown of PKCε using siRNA does not affect the SAC arrest in DLD-1 cells. ( a – d ) DLD-1 cells were treated with various SAC triggers and the fidelity of the SAC arrest was measured after loss of PKCε. ( a , b ) DLD-1 parental cells or DLD-1 PKCε M486A cells were treated with 100 μM Monastrol±20 nM NaPP1 ( a ) or with PKCε si1 ( b ) and time taken to transit through mitosis was assayed by time-lapse microscopy by monitoring cell rounding. Charts show the number of cells that maintain a mitotic arrest for more than 7 h. ( c , d ) DLD-1 parental cells or DLD-1 PKCε M486A cells were treated with taxol or ICRF193 as indicated±20 nM NaPP1 or with PKCε si1 and the time taken to transit through mitosis was assayed by time-lapse video microscopy by monitoring cell rounding. The graph shows the time taken to transit through mitosis as a cumulative frequency chart. For all live-cell experiments, n >30, all experiments repeated three times. Full size image PKCε regulation of SAC silencing Catenation appears to implement a PKCε-dependent delay to anaphase entry; we therefore sought to understand whether and how PKCε influences exit from the SAC under conditions of high catenation. We addressed this by determining whether key kinetochore components of the SAC came under PKCε control in catenation-challenged, transformed cells. Previous reports regarding kinetochore occupation during a catenation-triggered metaphase delay are mixed [4] , [29] ; however, in accordance with Toyoda and Yanagida [4] we find the level of Mad2 is below the lower detection limit, but observe retention of intense Bub1 and BubR1 staining in both the DLD-1 and HeLa cell models ( Supplementary Fig. 4a–c ). To assess the effect of inhibiting PKCε on localization of the SAC proteins remaining on the kinetochore, we arrested cells in metaphase using ICRF193 and added the PKCε inhibitor Blu577 (Compound 18 (ref. 50 )) for 20 min to establish whether PKCε plays a dynamic role in maintaining the checkpoint proteins on the kinetochore. Inhibition of PKCε causes acute loss of BubR1 and Bub1 from kinetochores of ICRF193-treated cells ( Supplementary Fig. 4a,b ). As biorientation is achieved at this point, this is consistent with a role for PKCε in triggering a delay to the release of BubR1 and Bub1 from the kinetochore when resolution of decatenation has not been achieved. PKCε inhibition modulates microtubule-dependent streaming of ZW10 The RZZ complex is known to play a role in mitotic exit and its depletion is associated with increased segregation errors resulting in multinuclear cells [51] . All of the components of the RZZ complex are localized to the kinetochore during prometaphase and bind to Zwint and Knl1 (refs 51 , 52 ). Our experiments indicate that both ZW10 and Zwilch change their steady-state localization when delayed by catenation in metaphase and become undetectable at the kinetochore ( Supplementary Fig. 5a,b ). Dynein is similarly reduced in cells delayed in response to ICRF193 but not nocodazole, suggesting a dependence on the mitotic spindle for this reduction in signal at the kinetochore ( Supplementary Fig. 5c ). In both of these conditions, Bub1 and Zwint remain attached to the kinetochore, indicating a selective change in the apparent binding affinity of the RZZ complex and not a general disassembly of kinetochore complexes. These altered properties suggest that under conditions of excess catenation, the RZZ complex and dynein may be actively removed from the kinetochore indicative of kinetochore microtubule attachments [53] . We investigated whether the RZZ complex was actively streaming on the spindle by using FLIP (fluorescence loss in photobleaching) to measure ZW10 kinetochore dynamics. Using a HeLa cell model, which stably expresses GFP-ZW10 at a level that does not perturb normal mitotic transition, we repeatedly bleached cytoplasmic GFP-ZW10 and measured its rate of loss from the kinetochore ( Fig. 5a,b ). As expected, cells that are delayed with metaphase catenation have a faster kinetochore ZW10 turnover rate than cells arrested using nocodazole ( Fig. 5c ). This indicates that stable microtubule attachments are made at this point and correlates with our finding that levels of Mad2 are low ( Supplementary Fig. 4c ) [53] . PKCε inhibition further decreases this half-life only in cells arrested using ICRF193, indicating that PKCε may have some input into the regulation of kinetochore stripping ( Fig. 5d ). 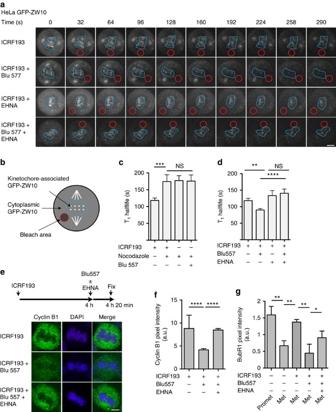Figure 5: ZW10 is actively stripped from the kinetochore when cells are delayed in metaphase using ICRF193 and this is modulated by both PKCε and dynein. (a–d) HeLa eGFP-ZW10 cells were arrested in metaphase with 10 μM ICRF193 or 250 nM nocodazole for 4 h and treated with either 100 nM Blu577 or 250 μM EHNA from the start of the video as indicated. Cells were then alternatively bleached (red circle) and imaged repeatedly, and the kinetochore intensity (blue dotted region) was fitted to a decay curve and corrected for intensity loss through imaging. (a) Representative stills from experiments. (b) Cartoon of experimental procedure. (c,d) Quantification of half-life measured during FLIP experiments as described above. Charts showing average ZW10 half-life. (n>20). (e–g) HeLa cells that are arrested in metaphase with ICRF193 have high levels of CyclinB1 and kinetochore BubR1. This is lost after inhibition of PKCε using Blu 557 in a dynein-dependent manner, suggesting stripping from the kinetochore. (e) Representative images. (f,g) Quantification of integrated pixel intensity measurements of CyclinB1 (f) or BubR1±s.e.m. (g) Chart shows mean of three experiments±s.e.m.,n>20 per condition per experiment. Scale bars, 5 μm. Figure 5: ZW10 is actively stripped from the kinetochore when cells are delayed in metaphase using ICRF193 and this is modulated by both PKCε and dynein. ( a – d ) HeLa eGFP-ZW10 cells were arrested in metaphase with 10 μM ICRF193 or 250 nM nocodazole for 4 h and treated with either 100 nM Blu577 or 250 μM EHNA from the start of the video as indicated. Cells were then alternatively bleached (red circle) and imaged repeatedly, and the kinetochore intensity (blue dotted region) was fitted to a decay curve and corrected for intensity loss through imaging. ( a ) Representative stills from experiments. ( b ) Cartoon of experimental procedure. ( c , d ) Quantification of half-life measured during FLIP experiments as described above. Charts showing average ZW10 half-life. ( n >20). ( e – g ) HeLa cells that are arrested in metaphase with ICRF193 have high levels of CyclinB1 and kinetochore BubR1. This is lost after inhibition of PKCε using Blu 557 in a dynein-dependent manner, suggesting stripping from the kinetochore. ( e ) Representative images. ( f , g ) Quantification of integrated pixel intensity measurements of CyclinB1 ( f ) or BubR1±s.e.m. ( g ) Chart shows mean of three experiments±s.e.m., n >20 per condition per experiment. Scale bars, 5 μm. Full size image Perturbation of dynein-mediated kinetochore stripping can be sufficient to prevent anaphase entry and thus we tested whether PKCε feeds into this pathway [54] . Erythro-9-3-(2-hydroxynonyl)adenine (EHNA) inhibits dynein ATPase activity and prevents cytoplasmic fluxing of dynein and its substrates [55] . We tested whether EHNA could prevent the kinetochore turnover of ZW10 in our system, to assess whether this was dominant over the exit from mitosis induced by PKCε inhibition. Interestingly, the decrease in half-life induced by PKCε inhibition can be prevented by inhibiting dynein ( Fig. 5d ). This indicates that mitotic exit triggered by PKCε inhibition is a dynein-dependent process. PKCε-mediated regulation of kinetochore SAC components As we can recover the effect of PKCε on ZW10 kinetochore turnover by dynein inhibition, we hypothesized that the mitotic exit triggered by PKCε inhibition may also be a dynein-dependent process. We found that in metaphase-delayed cells, acute inhibition of dynein does indeed block the degradation of cyclinB1 induced by acute PKCε inhibition in metaphase cells ( Fig. 5e–g ). We also investigated whether loss of BubR1 after PKCε inhibition is prevented, given that others have shown that this regulator can be stripped by dynein [22] , [54] , [56] . Interestingly, we find that the loss of BubR1 from the kinetochore after PKCε inhibition is also a dynein-dependent process ( Fig. 5g ). It is unclear whether the effect of inhibiting dynein in these assays is to directly prevent ZW10 streaming from the kinetochores or whether kinetochore microtubule binding is perturbed, because dynein is also known to play a role in stabilizing kinetochore microtubule interactions [56] . We see a small increase in prometaphase cells with dispersed metaphase plates, indicating that the cells transitioning from prometaphase to metaphase during the 20-min EHNA treatment do not fully congress to the metaphase plate and these cells have intense Mad2 signal ( Supplementary Fig. 4e ). This is in agreement with Varma et al. [56] who showed abnormal spindle equator orientation and oscillation of kinetochore pairs after dynein perturbation. We find that Mad2 is not stabilized on fully congressed metaphase kinetochores after EHNA treatment, indicating that these spindle attachments may be maintained ( Supplementary Fig. 4d,e ). This is in contrast to a short incubation with the microtubule depolymerizing agent nocodazole, which quickly causes recruitment of Mad2 to the kinetochores ( Supplementary Fig. 4f ). The evidence here defines a PKCε-dependent pathway as a conditional player in exit from the SAC that monitors appropriate sister chromatid decatenation (see Fig. 6 for working model). As part of this response, PKCε may trigger a resolution pathway as evidenced by an increase in catenation in mitosis after loss of PKCε activity. This catenation manifests as chromatin bridging and PICH-positive strands in anaphase. We further find that PKCε is required to trigger the metaphase delay in response to catenation, indicating that PKCε is required for a global response to metaphase catenation. Interestingly, it appears that this is particularly important in certain transformed cells, which have a weak G2 catenation checkpoint and therefore a heightened requirement for mitotic decatenation. This acquired, emergent behaviour suggests a transformed cell-specific vulnerability to PKCε inhibition. 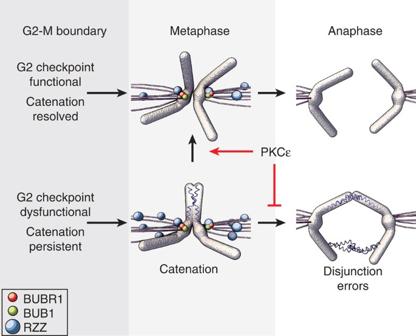Figure 6: Model of the PKCε-dependent metaphase catenation delay. There is a catenation checkpoint at the G2-mitosis boundary, which would normally trigger resolution of excess DNA catenation before entry into mitosis. If this process fails, as is the case in some transformed cells, there is a failsafe in metaphase, which is dependent on PKCε to both implement a delay and to trigger catenation resolution. This pathway is activated when there is persistent catenation after the spindle is fully aligned at the point of mitotic exit and is effected through a dynein-dependent modulation of the SAC. In cells with both an abrogated G2 catenation checkpoint and loss of PKCε, cells exit mitosis prematurely with disjunction errors caused by sister chromatid catenation. Figure 6: Model of the PKCε-dependent metaphase catenation delay. There is a catenation checkpoint at the G2-mitosis boundary, which would normally trigger resolution of excess DNA catenation before entry into mitosis. If this process fails, as is the case in some transformed cells, there is a failsafe in metaphase, which is dependent on PKCε to both implement a delay and to trigger catenation resolution. This pathway is activated when there is persistent catenation after the spindle is fully aligned at the point of mitotic exit and is effected through a dynein-dependent modulation of the SAC. In cells with both an abrogated G2 catenation checkpoint and loss of PKCε, cells exit mitosis prematurely with disjunction errors caused by sister chromatid catenation. Full size image PKCε plays an essential role in cytokinesis in some systems [34] , [35] , [57] . The anaphase bridging observed here correlates with cytokinesis failure, indicating that there may be a link between the two phenotypes. Close examination of the cytokinesis phenotype, using a very specific chemical genetic inhibitor, has shown that a cytokinesis defect can be induced by inhibition of PKCε once the cell is already in telophase. This suggests that although these phenotypes may be related, they can be triggered independently. The cytokinesis phenotype described previously may therefore be exacerbated by a failure to complete decatenation after PKCε knockdown and this may also explain the cell-type-specific penetrance of the phenotype [34] . The G2 catenation checkpoint is defective in a variety of different cancer cell lines [33] . We have shown that only cells with a leaky G2 catenation checkpoint enter mitosis with detectable basal catenation. These cells display a strong dependence on PKCε for the resolution of catenation in mitosis to avoid chromosome disjunction. We therefore propose that PKCε is working directly in mitosis to protect cells from anaphase entry with catenated sister chromatids, although we cannot rule out that PKCε has additional roles in other stages of the cell cycle. We show that normal (non-transformed) cells arrest robustly before mitosis when challenged by catenation, and that this arrest is not dependent on PKCε. We therefore suggest that this provides an explanation for the conditional requirement for PKCε in a subset of cell lines. The evidence indicates that PKCε is an apparently universal modulator of the metaphase catenation delay in the transformed cell lines tested and also in the non-transformed RPE cell line when a dependence is triggered using inhibitors of the G2 catenation checkpoint. This appears to operate predominantly independently of the arrest triggered by other perturbations that influence the SAC. However, there was one interesting outlier, where in HeLa cells the mitotic arrest induced by taxol shows an interaction with the PKCε-dependent pathway and was weakened on loss of PKCε. This was not the case in other cell lines tested. It is possible that a direct effect of taxol on topoIIa activity may contribute to this complexity [58] or perhaps that the PKCε pathway may be influencing a subtle taxol-inducible property to which HeLa cells are particularly sensitive. It has been shown by others that disruption of TopoIIa can interfere with tension sensing, which may provide some explanation for an interaction with the taxol-mediated arrest, although not for the discrepancy seen between different cell lines [4] , [59] . Indeed, a tension-mediated property may provide some basis for the mechanisms involved in detection of mitotic catenation and how this is mediated through the SAC. In support of a possible role for tension sensing, we and others show that the metaphase delay invoked by catenation is characterized by high levels of BubR1 and undetectable Mad2 at the kinetochore [4] . Acute inhibition of PKCε causes rapid loss of BubR1 from the kinetochore along with CyclinB1 degradation, indicating mitotic exit. This mitotic exit is dependent on dynein and is consistent with a role for PKCε in regulating the very last stages of disassembly of the mitotic checkpoint via regulation of dynein-dependent stripping of BubR1. CyclinB1 levels remain high and Mad2 levels low, suggesting that kinetochore BubR1 may be sufficient to impart a transient delay to APC activation in these circumstances, although we cannot rule out that low or transient kinetochore Mad2 is providing a diffusible APC inhibitor [11] . The RZZ complex and dynein are stripped from the kinetochore during the catenation delay, indicating that spindle attachments are formed during this time, and this is supported by the timely congression of the metaphase plate along with undetectable Mad2 on the kinetochore. It is not known whether kinetochore BubR1 is sufficient to inhibit the APC alone, although it is a strong candidate as it has a rapid kinetochore–cytoplasm exchange and is an inhibitor of the APC [12] , [60] . Notably, Huang et al. [61] show that retention of BubR1 on the kinetochore using a phosphomimetic mutant can delay anaphase onset. This is characterized by low levels of kinetochore Mad1 and a delay of around 2 h with full metaphase plate congression. This is similar to the delay shown here after inhibition of topoIIa. Exit from the SAC can be modulated by dynein- and RZZ complex-regulated stripping of checkpoint proteins from the kinetochore, allowing SAC silencing. We show evidence that the mitotic exit implemented by PKCε inhibition is a dynein-dependent process and show that the metaphase arrest stimulated by excess metaphase catenation is characterized by stripping of both the RZZ complex and dynein from the kinetochore along with ZW10. We show that PKCε can modulate the rate of ZW10 streaming by adding a PKCε-specific inhibitor during live-cell imaging, eliciting an increase in the rate of ZW10 streaming and showing that PKCε is playing an active role in mitosis. Reports regarding whether dynein-dependent streaming can regulate BubR1 kinetochore retention are mixed [22] , [62] . Others have shown that BubR1 is retained on the kinetochore when dynein-dependent stripping is disrupted by point mutations in Zwint [54] or by truncations of dynein itself [56] , showing dynein does regulate kinetochore BubR1 in some circumstances. Here we show loss of kinetochore BubR1 after PKCε inhibition before anaphase entry and show that this can be prevented by inhibiting dynein. On inhibition of dynein, we see no recovery of kinetochore Mad2, indicating that kinetochore BubR1 may be sufficient to impart the transient metaphase delay that we observe in response to catenation in metaphase. It is unclear precisely what triggers the metaphase response to catenation. TopoIIa appears to be intrinsically required for both resolution and catenation detection in both metaphase and G2. In both instances, deletion of the enzyme results in an abrogated catenation checkpoint and progression with non-disjunction to the next cell cycle phase [44] , [45] . ICRF193 is a class 2 topoismerase inhibitor that blocks topoIIa in a catalytically inactive state; it does not cause DNA damage directly as TopoIIa is retained in a conformation in which it cannot induce double-stranded breaks. However, this does not rule out DNA damage as a result of continued transit through the cell cycle with excess catenation, which may contribute to the mixed reports regarding the induction of DNA damage markers [45] , [63] . Inhibition with this drug triggers both the G2 and the mitotic checkpoint [29] , [45] . It therefore seems that the presence of TopoIIa in a particular catalytic state may be important for activation of both of the checkpoints. In accordance with this, Furness et al. [44] have isolated various catalytically inactive mutations of yeast top2 that differentially inactivate the mitotic catenation checkpoint, suggesting that checkpoint signalling is propagated through topoisomerase enzyme cycles and not through the DNA lesion itself [44] . Untangling this intriguing relationship with known functions of the SAC and also investigating what other replication stress-induced segregation perturbations may be detected and regulated in mitosis may prove to be important in our global understanding of the mechanisms used to protect cells from DNA damage and aneuploidy. Here we have identified PKCε as a conditional player in the mitotic checkpoint, which is engaged only in the context of metaphase catenation and serves to delay anaphase transition protecting from cell division failure ( Fig. 6 ). This conditional engagement provides a unique opportunity for intervention in those tumours dependent on PKCε due to a weak G2 catenation checkpoint [64] , [65] , [66] , [67] . The definition of this layer of SAC control opens up a promising avenue to new mitotic cancer therapeutics capitalizing on our growing understanding of the complexities involved in regulation of the cell cycle. Reagents All reagents, including Nocodazole, ICRF193, Colcemid, Taxol and Nocodazole, were purchased from Sigma Aldrich unless otherwise stated. ATM/ATR inhibitors were purchased from Calbiochem. BLU577 was kindly provided by Dr Jon Roffey, Cancer Research Technology, UK. Cell culture HeLa cells cultured in DMEM (Gibco)+10% FCS. For siRNA transfections, HiPerfect (Qiagen) was used according to the manufacturer’s recommendations; all siRNAs were used at a final concentration of 10 nM. Tetracycline-inducible 293 cell lines were generated using the T-Rex Flp In system (Invitrogen) according to the manufacturer’s instructions. To induce GFP–PKC expression, HEK 293 cells were cultured in DMEM containing 10% FCS and tetracycline (100 ng ml −1 ) for 24 h before assay. For siRNA transfections, HiPerfect (Qiagen) was used according to the manufacturer’s recommendations; all siRNAs were used at a final concentration of 10 nM. The following SmartPOOLs were purchased from Dharmacon: PKCε si1: Cat. D-004653-01 (5′-gggcaaagaugaaguauau-3′); PKCε si3: Cat. J-004653-08-0050 (5′-GACGUGGACUGCACAAUGA-3′); siBubR1Smartpool set of 4: Cat. LU-004101-00-0002 (5′-CAAUACAGCUUCACUGAUA-3′, 5′-GCAAUGAGCCUUUGGAUAU-3′, 5′-GAAACGGGCAUUUGAAUAU-3′, 5′-GAUGGUGAAUUGUGGAAUA-3′); siMad2 Smartpool set of 4: Cat. D-003271-05 (5′-GAAAGAUGGCAGUUUGAUA, 5′-UAAAUAAUGUGGUGGAACA-3′, 5′-GAAAUCCGUUCAGUGAUCA-3′, 5′-UUACUCGAGUGCAGAAAUA-3′); si topoIIa Smartpool set of 4: Cat. J-004239-09 (5′-GGUAACUCCUUGAAAGUAA-3′, 5′-GGAGAAGAUUAUACAUGUA-3′, 5′-GAUGAACUCUGCAGGCUAA-3′, 5′-CGAAAGGAAUGGUUAACUA-3′); siSgo1 Smartpool set of 4: Cat. D-015475-17 (5′-UGUGAAGGAUUUACCGCAA-3′, 5′-CAGCCAGCGUGAACUAUAA-3′, 5′-UGAAAGAAGCCCAAGAUAU-3′, 5′-CAUCUUAGCCUGAAGGAUA-3′). The remaining olionucleotides were purchased from Qiagen: PKCε si2: Cat. S100287784 (5′-cccgaccatggtagtgttcaa-3′); siControl: cat. 1027310 (5′-AATTCTCCGAACGTGTCACGT-3′). Microscopy For videomicroscopy experiments, cells were cultured on LabTek chambered coverglass slides (Nunc) in Leibovitz CO 2 -independent media (Gibco). A low light level inverted microscope (Nikon TE2000) imaging system equipped with a laminar-flow heater to maintain a constant temperature of 37±0.01 °C, a PlanFluor 40 × DIC lens and a Xenon lamp for fluorescent excitation. Images were taken using a high quantum efficiency charge-coupled device camera (Andor Ixon) every 4 min. Other images were taken using an inverted laser scanning confocal microscope (Carl Zeiss LSM 780) equipped with a × 63 Plan-APOCHROMAT DIC oil-immersion objective. For all experiments where live cell time lapse was carried out on individual cells, n >30, as this was the maximum number of cells that could be imaged in multiple position experiments with 3–4 min time points. Fast time points were required to capture all phases of mitosis and to capture transition time information. The experiments were repeated three times. For FLIP experiments, an inverted laser scanning confocal microscope (Carl Zeiss LSM 780) equipped with a × 63 Plan-APOCHROMAT DIC oil-immersion objective was used. HeLa cells that stably express GFP-ZW10 were used. Individual cells were alternatively imaged and bleached in a cytoplasmic 2-μm radius circle every 16 s, acquiring a 5 × 2 μm Z -stack to capture all kinetochores. The laser power was kept consistent between experiments at 65 W. Z -stack images were summed and time-lapse series were analysed using Metamorph software (Molecular Devices). Kinetochore-localized GFP-ZW10 intensity time courses were collected using Metamorph (Molecular Devices) and interpolated using Mathematica (Wolfram). The following exponential function was used: Ie+I1*Exp[− t / t 1], where Ie=background intensity, I1=initial intensity, t =time (s) and t1=time constant. Images were also collected with bleaching outside the cell to assess the effect of imaging to the half-life of GFP-ZW10. The mean of these values were used to correct the T1 values derived from FLIP experiments to achieve a more accurate representation of GFP-ZW10 half-life using the following function: T 1=( T c T 2)/T2−Tc), where T1=GFP-ZW10 time constant, T2=slow decay caused by imaging, Tc=sum of T1 and T2. T1 half-life values were obtained by multiplying these values by (1/ln(0.5)). ZW10 kinetics were measured for at least ten cells per condition and this sufficient to control for biological variability. For CLEM, cells were grown on photo-etched gridded coverslips and fixed in 4% paraformaldehyde in 0.1 M PBS. Cells of interest were identified and imaged using fluorescence and phase contrast microscopy after knockdown of PKCε using siRNA. Cells were then fixed in 2·5% glutaraldehyde/4% paraformaldehyde in 0.1 M Phosphate Buffer for 1 h. The samples were post-fixed in reduced osmium tetroxide, stained with tannic acid, dehydrated stepwise to 100% ethanol and embedded in epon. The cells of interest were relocated on the block face and serial sections (~70 nm) were cut using an Ultracut UCT ultramicrotome (Leica Microsystems UK), collected on formvar-coated slot grids and post-stained with lead citrate. Serial sections were viewed using a Tecnai G2 Spirit 120 kV transmission electron microscope (FEI Company) and an Orius charge-coupled device camera (Gatan UK). Immunofluorescence and immunoblotting For immunofluorescence experiments, cells were grown on 13 mm poly- L -lysine (Sigma-Aldrich)-coated glass coverslips and fixed with 4% paraformaldeyhyde/PBS for 15 min. Cells were then permeabilized with 1% Triton X-100 (Sigma Aldrich), blocked using 1% BSA (Sigma Aldrich) and probed using the following primary antibodies, all diluted at 1:100 in 1% BSA/PBS: rabbit anti-BubR1 (Cell Signaling Technology D32E8), sheep anti-Bub1 (ref. 68 ) (SB1.3) (courtesy of S. Taylor), mouse anti-cyclinB1 (Santa-Cruz Sc-245), mouse anti-phosphoH2A.X (Millipore JBW301) and mouse anti-PICH (Millipore 04-1540). For Triton X-100 pre-extraction assays, cells were grown on 13 mm coverslips and staining was carried out as above, except they were simultaneously fixed and permeabilized using 2% paraformaldeyhyde 1% Triton X-100/PBS for 30 min. The following primary antibodies were used in these assays: sheep anti-Bub1 (ref. 68 ) (SB1.3) (courtesy of S. Taylor), rabbit anti-Mad2 (Bethyl Laboratories A300-301A), mouse anti-ZW10 (AbCam ab53676), mouse anti-Zwilch (Sigma Aldrich C1C9), rabbit and Zwint (AbCam ab84367), mouse anti-PICH (Millipore 04-1540) and human anti-Centromere (ACA) (Antibodies Inc.15-234-0001). All coverslips were mounted using ProLong Gold with DAPI (Invitrogen). Immunoblotting was carried out by lysing samples using LDS sample buffer (Invitrogen) and resolving protein by SDS–PAGE using NuPAGE Bis-TRIS gradient gels (Invitrogen). Samples were then transferred to polyvinylidene difluoride membranes (Amersham) and probed using targeted antibodies and Luminata chemiluminescence detection system (Millipore). The following antibodies were used in these assays, all diluted at 1:1,000 in 1% BSA/PBS/0.05% TWEEN-20: rabbit anti-PKCε (Santa Cruz sc-214), mouse anti-topoIIa (Millipore Mab4197), mouse anti-alpha-tubulin (Sigma T5168), mouse anti-PICH (Millipore 04-1540), rabbit anti-Mad2 (Cell Signaling Technology D8A7) and mouse anti-BubR1 (NovisBio NB100-353BR1). Band densitometry was carried out using Image J software and normalized to a tubulin loading control. FACS analysis of G2 and mitotic cells To determine the permeability of the checkpoint, we added nocodazole to capture the cells that pass through the G2 checkpoint into mitosis. We measured the number of cells that were arrested in mitosis at the end of this assay by staining with propidium iodide to measure DNA content and an MPM-2 antibody to measure the number of cells in mitosis [69] . Cells were treated with various combinations of 1 μM nocodazole, 100 nM ATM inhibitor, 10 μM ATR inhibitor, 10 μM ICRF193 and 10 μM bleomycin for 24 h. Cells were fixed in ice cold 70% ethanol for 24 h and stained with 50 μg ml −1 propidium iodide and 100 μg ml −1 RNAase to analyse DNA content. Cells were then stained with a MPM-2 antibody that is directly conjugated to Alexa 633 (Millipore 16–220) for 2 h at room temperature and fluorescence intensity was measured using a using FACS Calibur (Becton Dickinson). This data was then analysed using the FlowJo software. Quantification of immunofluorescence images Imaging was carried out using Carl Zeiss LSM 780 confocal microscope equipped with a × 63 Plan-APOCHROMAT DIC oil-immersion objective and serial 1 μm Z-sections with a 1μm pinhole were taken to ensure full coverage of chromatin region. All image quantification was carried out using Metamorph image analysis software (Molecular Devices). Z -sections were summed and corrected for background signal (area with no cell). An inclusive threshold was then chosen to include all kinetochore signal in the positive control and applied to all images. Total integrated intensity for the chromatin region after thresholding was then measured for each cell. At least ten cells were measured for each condition and this is sufficient to control for biological variability. Catenation spread assay For measurement of metaphase catenation, cells were treated with siSgo1 for 24 h, followed by 1-h treatment with nocodazole to collapse the mitotic spindle, to aid spreading. Cells were collected by shaking off the mitotic cells and resuspended in a hypotonic solution of 75 mM KCl and incubated at 37 °C for 30 min to expand the cell. Cells were then resuspended in 3:1 methanol:acetic acid and fixed overnight at −20 °C. Cells were then spread onto clear slides by dropping from 1 m height. For assays where topoIIa was reintroduced, recombinant topo IIa (1 U μl −1 , TopoGen) was incubated in the hypotonic step where the cell membrane becomes hyperpermeable. The hypotonic buffer used here contained 5 mM Tris-Cl, pH 8.0, 75 mM KCl, 10 mM MgCl 2 , 0.5 mM ATP, 0.5 mM dithiothreitol. We confirmed by video-microscopy that there was no significant difference between the time that all samples had been arrested in mitosis at the start of the assay. Statistical tests In all cases where P -values are given an unpaired t -test was used. In the cases where the data includes more than two conditions, a one-way analysis of variance was used. Prism software (Graphpad) was used for all calculations. The level of statistical significance is represented as follows: n.s.= P >0.05, *= P ≤0.05, **= P ≤0.01, ***= P ≤0.001 and ****= P ≤0.0001. How to cite this article: Brownlow, N. et al. Mitotic catenation is monitored and resolved by a PKCε-regulated pathway. Nat. Commun. 5:5685 doi: 10.1038/ncomms6685 (2014).